Exploitation of desilylation chemistry in tailor-made functionalization on diverse surfaces Interface engineering to attain a uniform and compact self-assembled monolayer at atomically flat surfaces plays a crucial role in the bottom-up fabrication of organic molecular devices. Here we report a promising and operationally simple approach for modification/functionalization not only at ultraflat single-crystal metal surfaces, M(111) (M=Au, Pt, Pd, Rh and Ir) but also at the highly oriented pyrolytic graphite surface, upon efficient in situ cleavage of trimethylsilyl end groups of the molecules. The obtained self-assembled monolayers are ultrastable within a wide potential window. The carbon–surface bonding on various substrates is confirmed by shell-isolated nanoparticle-enhanced Raman spectroscopy. Application of this strategy in tuning surface wettability is also demonstrated. The most valuable finding is that a combination of the desilylation with the click chemistry represents an efficient method for covalent and tailor-made functionalization of diverse surfaces. Self-assembled monolayers (SAMs) on metal surfaces with desired physicochemical functions are of prime importance in the fields of organic and molecular electronics, sensors and protective coatings [1] , [2] , [3] , all of which benefit from the unique tunable structural properties of organic molecules. Owing to the crucial effect of surface morphology, stability and monolayer defects on the device efficiency [4] , [5] , there remains a pressing challenge in the interface engineering to form a stable, uniform and dense SAM on an atomically flat surface, which finally is an essential prerequisite for bottom-up device fabrications. In practice, many organic functional groups can be introduced to bind the molecules to the substrates for covalently modifying surfaces. The most popular approach to date mainly includes controlled chemisorption of thiols and electrochemical reduction of diazonium salts. The former has been applied on single-crystal electrodes such as Au [6] , [7] , [8] , Pt [9] and Pd [10] . However, it turns out that the degradation of the resulting SAMs remains a major limitation for further widespread applications in aqueous and ambient environments [7] , [11] . As a consequence, the latter method serves as an alternative strategy for the surface modification of Au, Pt and highly oriented pyrolytic graphite (HOPG) via the formation of highly stable covalent carbon σ-bonds on the surfaces [12] , [13] . However, it provides uncontrollable multilayer formation. Although a multilayer assembly offers abundant functional sites [14] , well-controlled homogeneity of the molecular monolayer is required for organic and molecular electronic devices [15] . In view of that, it clearly merits further studies to gain good control over the uniformity as well as stability of a wide range of functional SAMs. From another perspective, which comes from the field of molecular electronics, it has recently been demonstrated that molecules trapped between two gold electrodes by forming covalent Au – C σ-bonds display significantly higher conductance than those with thiol or other conventional anchoring groups [16] , [17] , [18] , [19] . This finding bears relevance while showing that the direct covalent Au–C bond formation leads to a strong electronic coupling because of an uninterrupted conjugation between the gold electrode and the molecule. Noteworthy studies along this line include the formation of an ultrastable SAM of N -heterocyclic carbines (NHCs) [20] and of highly ordered SAMs of alkynes on a Au(111) surface [21] . Finally, it is also worth noting that in contrast to the present understanding of surface modifications on gold electrodes and clusters [6] , little is known, however, about modifying other transition metal surfaces [6] , [9] , [10] , [22] , [23] , [24] . Thus, it is timely and highly desirable to develop a facile and versatile approach for the functionalization of a variety of surfaces. In order to lay emphasis on the aforementioned issues, we direct our attention towards the desilylation chemistry applied to in situ surface functionalization while forming covalent substrate – C σ-bonds. De facto and, quite advantageously, trialkylsilylacetylene reagents, as silyl-protected acetylenes, are widely used for transition metal-catalysed C–C bond formation reactions [25] , [26] . The desilylation with tetra- n -butylammonium fluoride (TBAF) has proven to be very powerful in acetylene chemistry because of its simple synthetic procedure, high efficiency and remarkable compatibility with different functional groups. As a beneficial outcome, a large variety of silyl-protected acetylenes, which are either commercially available or readily synthesized, allows access to diverse π-conjugated systems including small organic molecules and oligomers. Their general availability and ease of synthesis offer plenty of opportunities to substantially expand the surface chemical reactions on the basis of the desilylation chemistry. To further elaborate on this concept, a systematic study of functionalization at ultraflat single-crystal M(111) electrodes (M=Au, Pt, Pd, Rh and Ir, see Supplementary Fig. 1 and Supplementary Note 1 ) as well as at the HOPG surface with a series of ferrocene (Fc)-terminated trimethylsilyl (TMS)-protected oligo-(phenylene ethynylene) (OPE) molecules ( Supplementary Figs 2 and 3 ) was undertaken. The modified metal/carbon electrodes were characterized by cyclic voltammetry (CV), scanning tunnelling microscopy (STM) and shell-isolated nanoparticle-enhanced Raman spectroscopy (SHINERS) to gain insight into surface coverage, morphology and binding configuration. For the first time, we demonstrate herein that various metallic surfaces and, as a matter of fact, also carbon materials can be functionalized via desilylation chemistry. This study also provides examples to demonstrate the control of the surface functionality, for example, wettability, and most importantly the successful application of the click chemistry on surface. Thus, the present desilylation strategy promises to prepare tailor-made functional surfaces for their wider exploitation in molecular electronics, catalytic and biotechnological processes, and electrochemistry. Modification/functionalization at various surfaces We present the concept for metal and HOPG surface modifications involving the formation of a metal–carbon (M–C) or C–C covalent bond via in situ desilylation of silyl-protected acetylene derivatives using TBAF ( Fig. 1a ). This new approach has been examined by both electrochemical and spectroscopic methods. The characterization by CV demonstrates the grafting of ferrocene-terminated OPE molecules 1–3 with varied lengths, for example, on the Au(111) surface ( Fig. 1b,c ). Thereby, we identified a single pair of current peaks (P1, P1′), which is attributed to the ferrocene oxidation and ferrocenium reduction ( Fig. 1c ). The anodic and cathodic peak currents I a and I c scale linearly with the scan rate ( Supplementary Fig. 4 ), indicating a surface-confined electron-transfer reaction. The peak-to-peak separation does not exceed 20 mV. All these observations confirm the attachment of Fc-terminated molecules on the Au(111) surface. The slightly increased half-peak width going from 1 to 2 indicates repulsive interactions among oxidized Fc + moieties. A broader oxidation peak with a shoulder (P2) was observed for 3 , which is the longest molecule in our study. Similar phenomena are also observed in aqueous HClO 4 solution (see Supplementary Fig. 5 and Supplementary Note 2 ). The peak asymmetry caused by the appearance of an additional shoulder can be explained by subsequent oxidation of ferrocene moieties next to ferrocenium ions that are formed at more negative potential at peak P1. The shoulder P2 is absent when coverage is small (for example, <35% for 1 /Au(111)). Considering the packing arrangement within the SAM and approximating the ferrocene moieties as spheres with a diameter of 0.66 nm, a theoretical maximum coverage of 1–3 on Au(111) will have a density of 4.5 × 10 −10 mol cm −2 (100%; refs 27 , 28 ). The integration of redox peaks gives an increasing surface coverage of (32.9±2.0)%, (41.1±2.2)% to (51.3±2.0)% for 1 , 2 and 3 , respectively ( Supplementary Figs 6 and 7 ). This result might be accounted for by the relative solubility of 1 – 3 in tetrahydrofuran (THF). Increasing the length of the OPE chains drastically affects the solubility. Longer OPE molecules with a higher tendency to aggregate are less soluble; therefore, they are expected to have higher free energy in solution, but larger affinity for adsorption [28] . The observed average surface coverage of ~40% is comparable to those for Au electrodes modified with the same Fc-terminated molecules through Au–S bonds [27] , [28] . 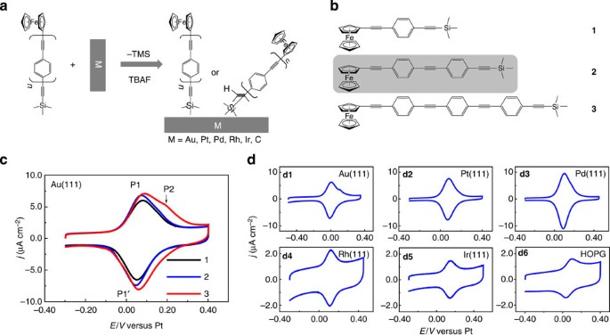Figure 1: Covalent binding of Fc-terminated OPE molecules at surfaces of different single crystalline materials. (a) Schematics of M–C covalent bond formation. (b) Molecules under study. (c) Cyclic voltammograms of1–3modified Au(111) surfaces in HMIm-PF6ionic liquid with scanning rate 50 mV s−1. (d) Steady-state cyclic voltammograms of2-modified Au(111) (d1), Pt(111) (d2), Pd(111) (d3), Rh(111) (d4), Ir(111) (d5) and HOPG (d6) in HMIm-PF6ionic liquid with scanning rate 50 mV s−1. Figure 1: Covalent binding of Fc-terminated OPE molecules at surfaces of different single crystalline materials. ( a ) Schematics of M–C covalent bond formation. ( b ) Molecules under study. ( c ) Cyclic voltammograms of 1–3 modified Au(111) surfaces in HMIm-PF 6 ionic liquid with scanning rate 50 mV s −1 . ( d ) Steady-state cyclic voltammograms of 2 -modified Au(111) ( d1 ), Pt(111) ( d2 ), Pd(111) ( d3 ), Rh(111) ( d4 ), Ir(111) ( d5 ) and HOPG ( d6 ) in HMIm-PF 6 ionic liquid with scanning rate 50 mV s −1 . Full size image Furthermore, the versatility of the actual strategy was explored on other single-crystal metal electrodes such as Pt, Pd, Rh and Ir ( Supplementary Figs 4 and 6 ). The CVs of 2 -modified Pt(111) and Pd(111) electrodes ( Fig. 1d2 ) display symmetric, well-defined current peaks. Since less is known about SAM functionalization at Rh(111) and Ir(111) surfaces, it appears quite promising that the desilylation chemistry leads also to a surface coverage in the range of 5–6% ( Fig. 1d4 , Table 1 ). Table 1 Absolute ( Γ ) and normalized surface coverages of 2 bonded to different single-crystal surfaces. Full size table Undoubtedly, carbon is one of the most promising materials for future organic and molecular electronics [29] , [30] . Grafting a uniform monolayer of functional molecules through a covalent C–C bond to carbon substrates such as HOPG, graphene or carbon nanotubes remains a challenge. To date, the most popular strategy involves reduction of diazonium salts on the surface [31] , [32] , [33] , [34] , [35] , including a recent effort using TMS protection groups for better control of the molecular assembly [34] . To assess whether the aforementioned TMS-cleavage concept is applicable to an HOPG surface as well, we tested its modification through grafting of an OPE-type molecule on it (see Supplementary Fig. 8 and Supplementary Note 3 ). Figure 1d6 shows the CV of the HOPG surface modified by 2 according to the same procedure as for the metal electrodes. Integration of the redox peaks (with correction of double-layer charging) yields a surface coverage of (0.26±0.04) × 10 −10 mol cm −2 , corresponding to a normalized surface coverage of (5.8±0.9)% ( Table 1 ). SHINERS and STM studies The question that now arises concerns the binding motif of the terminal alkyne on the surface and why the surface coverage varies significantly on different surfaces. A helpful indication is provided by SHINERS experiments [36] . As illustrated in Fig. 2a , a sandwich structure of substrate| 2 |Au@SiO 2 was created by depositing a submonolayer of Au@SiO 2 nanoparticles (NPs) on a SAM-modified surface for Raman enhancement. The Raman spectrum of the 2 -modified Au(111) surface (d-2) exhibits vibrational peaks, which are coincident with those of 2 in the solid state (for example d-1, see Supplementary Note 4 ), suggesting that the OPE molecules 2 remain intact after being grafted on the Au(111) surface ( Fig. 2d ). Significantly, the disappearance of the TMS vibration band at 1,457 cm −1 ( e2 , see Supplementary Fig. 9 and Supplementary Note 4 ) demonstrates the cleavage of the TMS group. The most direct evidence for the formation of Au−C σ-bonds arises from the appearance of a new band at 397 cm −1 ( e1 ), which is characteristic of a Au–C-stretching mode [37] , indicating that the resultant alkynylide binds to the Au(111) surface forming the Au−C σ-bond [19] . Consequently, one also observes the appearance of the new vibration mode at 2,001 cm −1 ( e4 ), which is assigned to the stretching mode of the −C≡C− unit that is covalently bound to the Au(111) surface. This assignment is firmly supported by the fact that the relative ratio of integrated intensity of −C≡C− stretching band v 1 (covalently linked to the gold surface) to v 2 (free −C≡C− stretching band) increases linearly, approximately from 1:1 to 1:3 with respect to increasing the repeating unit ( n ) of the OPE linker from 1 to 3, as demonstrated nicely in Fig. 2f . These observations are consistent with our previous report on the covalent Au–C (alkynylide) σ-bond formation [19] . 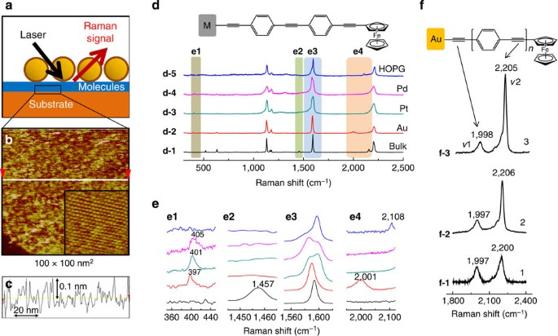Figure 2: SHINERS of SAM-modified surfaces. (a) Schematics of SHINERS configuration. (b) STM image showing the surface morphology of2-modified Au(111) surface. Imaging conditions: bias=300 mV, tunnelling current=100 pA. Inset: STM image shows the atomic resolution of Au(111) (1 × 1) atoms underneath the2SAM with extreme imaging conditions of low bias voltage (10 mV) and high setpoint of tunnelling current (3 nA). (c) Cross-section profile along the white line inbshowing the apparent height of the monolayer. (d) Raman spectra of2in the solid state (d-1) and as a monolayer of2on Au(111) (d-2), Pt(111) (d-3), Pd(111) (d-4) and HOPG (d-5) surfaces. (e1–4) Magnifications of the interesting regions as indicated ind. (f) Raman spectra of1(f-1),2(f-2) and3(f-3) on Au(111) within the specified frequency regions of the C≡C stretching mode. Figure 2: SHINERS of SAM-modified surfaces. ( a ) Schematics of SHINERS configuration. ( b ) STM image showing the surface morphology of 2 -modified Au(111) surface. Imaging conditions: bias=300 mV, tunnelling current=100 pA. Inset: STM image shows the atomic resolution of Au(111) (1 × 1) atoms underneath the 2 SAM with extreme imaging conditions of low bias voltage (10 mV) and high setpoint of tunnelling current (3 nA). ( c ) Cross-section profile along the white line in b showing the apparent height of the monolayer. ( d ) Raman spectra of 2 in the solid state ( d-1 ) and as a monolayer of 2 on Au(111) ( d-2 ), Pt(111) ( d-3 ), Pd(111) ( d-4 ) and HOPG ( d-5 ) surfaces. ( e1–4 ) Magnifications of the interesting regions as indicated in d . ( f ) Raman spectra of 1 ( f-1 ), 2 ( f-2 ) and 3 ( f-3 ) on Au(111) within the specified frequency regions of the C≡C stretching mode. Full size image Comparative Raman experiments with 2 -modified Pt(111) and Pd(111) surfaces also exhibit a M–C stretching mode at ~400 cm −1 ( e1 ). However, the band around 2,000 cm −1 , characteristic of the −C≡C− stretching mode of the alkynylide attached to the surface, was not observed ( e4 ). In contrast, the splitting of the Raman band at 1,586 cm −1 in the region of C=C stretching in addition to the feature of benzene ring was observed for 2 on both Pt and Pd surfaces ( e3 ). This phenomenon is also reproducible on 3 (see Supplementary Fig. 10 and Supplementary Note 5 ), and is probably because of the formation of newly surface-bounded C=C through the rehybridization of C≡C when attached to the catalytically active Pt/Pd surface. The similar rehybridization from sp to sp 2 was also observed for acetylene when adsorbed either on Pt and Rh surfaces under electrochemical conditions [38] or on Rh(111) in UHV [39] . Such rehybridization of the C≡C bond is generally explained by the Dewer–Chatt–Duncanson model [40] . In this structural model, the filled acetylene π-orbital overlaps with an empty metal d-orbital, while the empty π*-orbital overlaps with a filled metal d -orbital. On the basis of our Raman observations, we propose that the same rehybridization process from sp to sp 2 also happens to the actual alkyne-terminated Fc molecules. The 2 -modified HOPG (d-5) has similar spectral features as the corresponding 2 -modified Au(111), except for an increase in the vibrational frequency of the surface-bounded C≡C stretching mode from 2,001 cm −1 (on Au) to 2,108 cm −1 . This result suggests that the generated alkynylide binds less strongly to the HOPG surface than to gold. Nevertheless, the C≡C stretching frequency shows a shift of 100 cm −1 upon binding to the HOPG surface. Given by the fact that step edge sites of the HOPG surface contain different kinds of functional groups such as anhydride, lactone, semiquinone and so on [41] , [42] , [43] , we conclude that the alkynylides undergo a nucleophilic addition to carbonyl groups at the step edge sites leading to the formation of propargyl alcohols. This binding motif is also supported by the STM image showing the preferential adsorption of 2 on the step edge sites of the HOPG surface ( Supplementary Fig. 11 ). Consequently, the 2 -modified HOPG (d-5) shows the C≡C stretching mode at similar frequency to propargyl alcohols. Figure 2b shows a representative STM image of 2 -modified Au(111) revealing an island/vacation-free monolayer. As expected, no highly ordered Fc SAM was found because of the rigidity of Fc-terminated molecular wires [27] . Notably, the TMS-cleavage approach provides the preservation of an intact Au(111) substrate ( Supplementary Fig. 12 ), in contrast to restructuring the gold surface leading to the etch pits as reported on thiol- [27] and NHC-based [20] SAMs. The corrugation height of the terraces in STM images does not exceed 0.15 nm, which indicates the absence of multilayer formation. Furthermore, a close inspection with a high tunnelling current (3 nA) and low bias (10 mV) shows an atomically flat Au(111) surface underneath the SAM ( Fig. 2b inset). The findings herein represent a unique opportunity to fabricate highly efficient top contacts on the atomically flat surface for molecular electronic devices. Electrochemical stability of the modified surfaces To evaluate the stability of the resulting SAMs, CV experiments of 2- modified Au(111) were carried out with potential cycling in the potential window of ferrocene oxidation/ferrocenium reduction for more than 100 h. As illustrated in Fig. 3a , the evolution of CVs shows that the intensity of the oxidation peak decreases gradually over 10,000 cycles at a scan rate of 50 mV s −1 . The normalized surface coverage (first cycle=100%) with respect to every 1,000 cycles is plotted in the right-hand y axis of Fig. 3a . The coverage drops more abruptly over the first 1,000 cycles, and then decreases only slightly during the subsequent 9,000 cycles. It is evident that ~55% of compound 2 was kept on the surface after 10,000 cycles, indicative of stable SAM formations on Au(111) surfaces via the TMS-cleavage approach. A similar experiment on Pt(111) showed less than 7% loss in surface coverage over 3,000 cycles (see Supplementary Fig. 13 and Supplementary Note 6 ). The electrochemical potential window of 2 on Au(111) were further evaluated in aqueous electrolytes of HClO 4 for oxidative desorption and NaOH for reductive desorption ( Fig. 3b ), respectively. The reductive desorption current peak P red is observed at ~−0.95 V (versus SCE) and the oxidative desorption peak P oxi at ~1.21 V (versus SCE). The resultant wide potential window of ~2.20 V is similar to that for thiol-based organic molecules assembled on gold surfaces [44] ; however, the P red is negatively shifted by 0.50 V in comparison with the NHC on a Au(111) surface [20] . 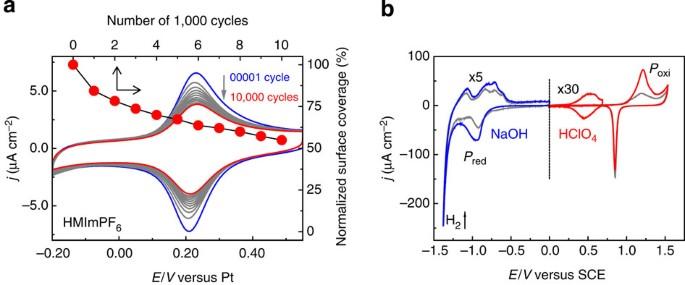Figure 3: Stability of the 2-modified Au(111) surface. (a) Left axis: CVs of continuous potential cycling in HMIm-PF6at a scan rate of 50 mV s−1of a monolayer of2-modified Au(111) surface, shown in the sequence of one thousand cycles; right axis: normalized evolution of surface coverage of2. (b) CVs showing the potential window of2-modified Au(111) in aqueous electrolyte of NaOH (blue curve, left half panel) and HClO4(red curve, right half panel) at a scan rate of 10 mV s−1. The blue and red curves indicate the first potential cycle and the grey curves represent the subsequent second cycle. Figure 3: Stability of the 2-modified Au(111) surface. ( a ) Left axis: CVs of continuous potential cycling in HMIm-PF 6 at a scan rate of 50 mV s −1 of a monolayer of 2 -modified Au(111) surface, shown in the sequence of one thousand cycles; right axis: normalized evolution of surface coverage of 2 . ( b ) CVs showing the potential window of 2 -modified Au(111) in aqueous electrolyte of NaOH (blue curve, left half panel) and HClO 4 (red curve, right half panel) at a scan rate of 10 mV s −1 . The blue and red curves indicate the first potential cycle and the grey curves represent the subsequent second cycle. Full size image Applications in surface functionalization In the following it will be demonstrated that the strategy of desilylation chemistry does indeed facilitate a wide range of surface functionalization. First, we direct attention towards the control of surface wettability by covalently tethering molecules with hydrophobic or hydrophilic tail groups at the Au(111) surface. Specifically, the hydrophobicity/hydrophilicity of the surface was tuned by termination with molecules bearing either a fluorocarbon chain ( 4 ) or polyoxyethylene chains ( 5 ), respectively ( Fig. 4a,b ). Water contact angle measurements were carried out on 4- and 5- modified Au(111) surfaces, resulting in the contact angle value of 95±1° and 67±1°, respectively. The contact angle of 95° for 4 /Au(111) is in good agreement with the value of 95±3° measured for an analogous fluorosurfactant physisorbed on Au(111) (ref. 45 ); this surfactant holds a similar length of the fluorocarbon chain with a fluoromethyl end group. In contrast, while molecules with hydrophilic polyoxyethylene chains ( 5 ) were employed, although terminated with methyl groups, a smaller contact angle of 67±1° was observed. 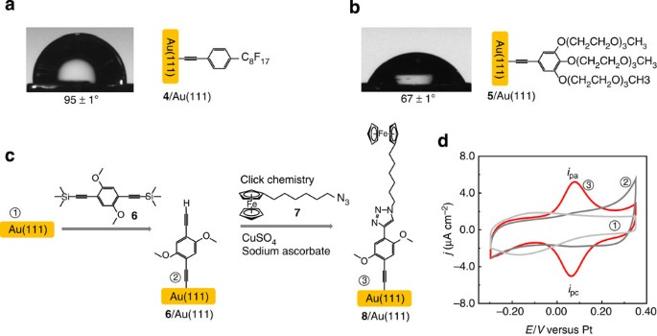Figure 4:Hydrophobicity/hydrophilicity tuning and on-surface click chemistry. (a,b) Contact angle of ultrapure water droplet on (a)4-and (b)5-modified Au(111) surface (denoted as4/Au(111) and5/Au(111), respectively). (c) Schematics of the click chemistry reaction at a surface. (d) Cyclic voltammograms of the three corresponding electrodes (1–3) as indicated incin HMIm-PF6at a scan rate of 50 mV s−1. Figure 4: Hydrophobicity/hydrophilicity tuning and on-surface click chemistry . ( a,b ) Contact angle of ultrapure water droplet on ( a ) 4- and ( b ) 5- modified Au(111) surface (denoted as 4 /Au(111) and 5 /Au(111), respectively). ( c ) Schematics of the click chemistry reaction at a surface. ( d ) Cyclic voltammograms of the three corresponding electrodes (1–3) as indicated in c in HMIm-PF 6 at a scan rate of 50 mV s −1 . Full size image To further elaborate on the concept of the desilylation chemistry, we employed the click chemistry for modulating the surface functionalities [34] , [46] . As shown in Fig. 4c , first the alkyne-terminated Au(111) surface, 6 /Au(111), was prepared by the same method of desilylation as for 1–3 on Au(111). This step was followed by a click chemistry reaction, namely Cu(I)-catalysed Huisgen 1,3-dipolar cycloaddition [47] , with the azide-terminated ferrocene molecule 7 , which resulted in the expected product 8 /Au(111). CV was performed to test and quantify the as-formed new monolayer. The red curve in the cyclic voltammogram of Fig. 4d displays a well-defined symmetric redox signal of ferrocene/ferrocenium, characteristic of immobilized Fc moieties. The redox peaks exhibit a narrow peak-to-peak separation of 15 mV, and the peak height of both the oxidative ( i pa ) and the reductive ( i pc ) signals display linear dependence on potential scan rate ( Supplementary Fig. 14 ), clearly indicating surface-bounded ferrocene molecules. On the basis of integration of the anodic peak, a surface concentration of grafted ferrocene moieties is estimated to be 1.3 × 10 −10 mol cm −2 , which is around two-third of the coverage of 2 on Au(111). Control experiments were carried out on both, only 6 -modified Au(111) and bare Au(111) electrodes showing the lack of the characteristic redox current signal of ferrocene/ferrocenium (light-grey and grey curves in Fig. 4d ). All these results unambiguously evidence the successful demonstration of the combination of the desilylation and the click chemistry on surface. We have developed a facile, effective and versatile strategy for surface modification/functionalization on various material surfaces by fluoride-induced desilylation chemistry. Molecular self-assembly under ambient conditions can be performed within 15 min, leading to relatively high surface coverages. The formation of surface covalent bonds is unambiguously confirmed by detailed analyses of CV, STM and SHINERS. Important applications of this approach in tuning surface wettability and functionalization by click chemistry have been demonstrated. Beyond these results, this work demonstrates a simple, versatile and robust platform for various surface modifications/functionalizations. Current efforts move towards determining the mechanisms for different binding motifs of the terminal alkynes on catalytically active surfaces. Given the versatility and availability of widely used TMS-terminated molecules, it is envisaged that the desilylation chemistry can be used to create a wide range of exceptionally stable SAMs with specific functions on various metal and carbon surfaces for the elaboration of new materials with high added values of optical and electrical properties. Chemicals and organic synthesis Details of synthesis and characterization of the studied molecules are summarized in the Supplementary Methods . THF (HPLC grade) and 1-hexyl-3-methylimidazolium hexafluorophosphate (HMIm-PF 6 ) ionic liquid were purchased from Sigma Aldrich. The HMIm-PF 6 was pumped (10 −6 mBar) together with molecular sieve at elevated temperature (85 °C) overnight before using. Sample preparation The sample preparation was performed using Clavilier-type half-bead single-crystal electrodes (~2 mm diameter). The characterization of single-crystal electrodes by cyclic voltammograms are summarized in Supplementary Fig. 1 , indicating the high quality of single-crystal(111) surfaces. The electrodes were annealed in a butane-air flame for ~2 min and cooled down to room temperature in an Ar atmosphere for Au(111), Pd(111) and in Ar+H 2 mixture for Pt(111), Rh(111) and Ir(111). The freshly annealed electrodes were immersed in a freshly prepared mixture of 20 μl THF solution containing 1 mM molecule and 20 μl solution of 2 mM TBAF in THF at room temperature for 15 min. Afterwards, the electrodes were rinsed copiously by THF to remove the physisorbed species, and then dried under Ar flow and finally transferred to electrochemical, STM or Raman cell for measurements. The same procedure as described above for metal single-crystal electrodes was applied for the freshly cleaved HOPG electrode. On-surface click chemistry CuSO 4 /H 2 O (1 ml, 3 mM) was mixed with 1 ml of 7 /THF (3 mM), deaerated by Ar gas for 10 min. The 6- modified Au(111) electrode was immersed into the mixed solution. Sodium L-ascorbate/H 2 O (1 ml, 3 mM) was added into the mixed solution drop by drop under Ar atmosphere. The as-prepared 6 -modified Au(111) electrode was kept in solution for 2 h with continuous Ar bubbling. Afterwards, the electrode was removed from solution, and rinsed by THF and water in sequence. The electrode was immersed in 10 mM EDTA solution for 15 s, rinsed with water, immersed in 1 M NH 3 /H 2 O for 15 s and rinsed with water. This process of immersing the electrode subsequently in EDTA and NH 3 /H 2 O solutions was repeated two times more in order to remove copper residues. The electrode was dried under Ar flow and was ready for electrochemical measurements. Cyclic voltammetry Electrochemical measurements were performed with an Autolab PGSTAT 30 (Eco Chemie, the Netherlands). A custom-designed, single-compartment glass cell was used for voltammetric measurements in ionic liquid. This specially designed cell allows using the volume of working solution down to ~100 μl and enables keeping inert gas atmosphere inside. Pt wires were used as the counter and quasi-reference electrodes. A two-compartment electrochemical cell was used for the CV measurements in aqueous electrolytes, with a Pt wire as the counter electrode and a reversible hydrogen electrode as the reference electrode. A working electrode was brought to the contact with an electrolyte in a hanging meniscus configuration under a certain potential, at which the Fc was in the neutral form. All CV measurements were carried out under Ar atmosphere. STM experiments A Nanoscope E (Digital Instruments) was used for STM imaging measurements. The measurements were carried out in Ar atmosphere in a constant-current mode. The STM tips were prepared by mechanical cutting of the Pt–Ir wire (80/20%, 0.25 mm diameter, Goodfellow). Raman spectroscopy We employed SHINERS in M(111)|molecule|Au@SiO 2 -NP sandwich structures. The ~55-nm Au NPs obtained by a citrate reduction method were further coated with a pinhole-free thin silica film (thickness ~2–3 nm). Details were summarized in the Supplementary Methods . Raman experiments were performed with a HR800 confocal Raman spectrometer (Horiba JY, France). The excitation wavelength was 632.8 nm from a He–Ne laser. A 50-times magnification long-working-distance (8 mm) objective was used to focus the laser on the sample surface and to collect the scattered light in a backscattering geometry. The power on the sample was ~1 mW. Contact angle measurements Contact angles were measured with a EasyDrop Standard (KRÜSS GmbH, Hamburg, Germany). The experiments were performed under ambient conditions by using Milli-Q water (18.2 MΩ). How to cite this article: Fu, Y. et al . Exploitation of desilylation chemistry in tailor-made functionalization on diverse surfaces. Nat. Commun. 6:6403 doi: 10.1038/ncomms7403 (2015).